A photoconvertible fluorescent reporter to track chaperone-mediated autophagy Chaperone-mediated autophagy (CMA) is a selective mechanism for the degradation of soluble proteins in lysosomes. CMA contributes to cellular quality control and is activated as part of the cellular response to different stressors. Defective CMA has been identified in ageing and different age-related diseases. Until now, CMA activity could only be measured in vitro using isolated lysosomes. Here we report the development of a photoconvertible fluorescent reporter that allows monitoring of CMA activity in living cells. Activation of CMA increases the association of the reporter with lysosomes which can be visualized as a change in the intracellular fluorescence. The CMA reporter can be utilized in a broad variety of cells and is suitable for high-content microscopy. Using this reporter, we find that levels of basal and inducible CMA activity are cell-type dependent, and we have identified an upregulation of this pathway in response to the catalytic inhibition of the proteasome. Maintenance of a stable and functional cellular proteome requires continuous monitoring, repair and renewal of individual proteins [1] . Chaperones and two proteolytic systems, the ubiquitin/proteasome system and lysosomes, contribute to protein quality control in all cells. Degradation of intracellular proteins by lysosomes or autophagy can be attained through at least three different mechanisms: macroautophagy, microautophagy and chaperone-mediated autophagy (CMA) [2] . In the first two types of autophagy, proteins are delivered to the lysosomal lumen confined in vesicles that form de novo in the cytosol or by invaginations at the lysosomal membrane. In contrast, in CMA, single individual proteins are translocated across the lysosomal membrane [3] . Protein substrates for CMA bear in their amino-acid sequence a pentapeptide, biochemically related to KFERQ, which is recognized by the cytosolic chaperone of 70 kDa, hsc70 (ref. 4 ). The chaperone/substrate complex is targeted to lysosomes, where it binds to the lysosome-associated membrane protein type 2A (LAMP-2A), which then organizes into a multimeric complex required for substrate translocation [5] , [6] . Unfolding of the substrate protein, probably by chaperones at the lysosomal membrane, occurs before the substrate can cross the lysosomal membrane [7] assisted by a form of hsc70 resident in the lysosomal lumen (lys-hsc70). Once inside lysosomes, substrates are rapidly degraded by the luminal proteases. Some level of CMA activity can be detected under basal conditions in tissues such as liver, kidney, brain and in different cell types in culture, but cells maximally activate this pathway in response to stress [3] . CMA is upregulated during prolonged nutritional deprivation to provide amino acids through the degradation of proteins unnecessary under those conditions [8] . Oxidants, pro-oxidants and protein-denaturing toxins also elicit activation of CMA, which selectively removes the damaged proteins from the cytosol [9] , [10] . Compromised CMA leads to intracellular accumulation of oxidized and aggregated proteins and reduces cellular survival during stress [11] . In fact, the described decline of CMA activity with age may contribute to the increased susceptibility of old organisms to stress. Thus, we have previously shown that if CMA activity is preserved until late in life in livers of transgenic mice, they show significantly reduced levels of damaged proteins, better cellular homeostasis, higher resistance to stress and improved organ function than wild-type litter mates [12] . Reduced CMA activity in ageing may aggravate the progression of some age-related disorders such as neurodegenerative diseases and diabetes. In some of these disorders, such as Parkinson's disease or certain tauopathies, the pathogenic proteins that accumulate in the affected cells exert a direct toxic effect on CMA [13] , [14] , [15] . It is likely that alterations in CMA could contribute to the pathogenesis of other protein-conformational disorders. A major current limitation in the study of CMA physiology and the involvement of CMA failure in different disorders is the difficulty in monitoring CMA in intact cells. Current measurement of CMA requires using in vitro systems with isolated lysosomes in which each of the steps of CMA can be reproduced [16] . Although these systems have contributed to a large extent to our current understanding of this autophagic pathway, they require amounts of cells unattainable for primary differentiated and no-longer dividing cultured cells such as neurons or cardiomyocytes, and do not allow for the differentiation of CMA activity among the different cell types in a given tissue. To overcome these limitations and to be able to monitor CMA in intact cells, we have developed a photoconversion-based fluorescence method to image and quantify CMA activity in living cells. Introduction of a KFERQ-related motif into monomeric fluorescent proteins convert them into CMA substrates, which once targeted to lysosomes, highlight these compartments. The use of photoactivable proteins allows measurement of the dynamics of association and degradation of the reporter fluorescent protein in lysosomes through CMA. Using this novel fluorescent CMA reporter, we have found that basal and inducible levels of CMA activity are cell-type-dependent and have identified a previously unknown cross-talk between CMA and the proteasome. Development of a photoconvertible CMA reporter protein Fluorescent proteins have been used to monitor the activity of different intracellular proteolytic systems [17] , [18] , [19] , [20] . This often requires introducing a modification that targets the fluorescent protein to the proteolytic system of interest, and the analysis of either the association of the reporter with the degradative compartment or its cellular accumulation, when the proteolytic system is blocked. Taking advantage of the fact that attachment of the pentapeptide motif KFERQ to a given protein facilitates its degradation by CMA when this pathway is activated [4] , we used the first twenty-one amino acids of ribonuclease A, the first protein identified as a CMA substrate, that include the KFERQ motif, to generate cytosolic fluorescent proteins amenable for CMA degradation. Although delivery of these proteins to lysosomes by hsc70 should highlight this compartment as fluorescent puncta, our first attempts to visualize the degradation of a KFERQ-bearing enhanced green fluorescent protein (KFERQ–EGFP) using this approach failed, because of the intrinsic characteristics of CMA. As for any other CMA substrate [7] , translocation of KFERQ–EGFP to lysosomes is preceded by its complete unfolding and, with it, the loss of its fluorescence. Consequently, at any given time, the only lysosomal KFERQ–EGFP visible is the one bound to the lysosomal membrane but not yet translocated, and this amount is often too small to outline lysosomes against the cytosolic protein that fluoresce with the same properties. To overcome this limitation, we introduced the KFERQ-motif in a monomeric photoconvertible fluorescent protein, the photoswitchable cyan fluorescent protein [17] (PS-CFP2) ( Fig. 1a,b ). Photoconversion allows for following the lysosomal association of only the subset of this reporter converted to another fluorescence state, which exhibits different excitation and emission spectra ( Fig. 1c ). In this case, the protein synthesized after the photoconversion will be in the original fluorescence state (cyan) whereas the pool of protein present at photoconversion will fluoresce in green, allowing thus easy visualization of the green fluorescence puncta by decreasing this fluorescence in the cytosolic background. This procedure also permits measuring the degradation of the reporter as the decay in the levels of the photoconverted pool separately from its synthesis and without having to block CMA or lysosomal proteolysis. Inhibition of protein synthesis affects rates of protein degradation, and blockage of CMA results in compensatory changes in the activity of other proteolytic systems [11] , which has previously made it difficult to assess the contribution of CMA to degradation under normal physiological conditions. An added advantage of the use in our study of this latest generation of fluorescent proteins is that they preserve their monomeric features in cells [17] , preventing thus the non-selective lysosomal delivery of oligomeric and aggregates of fluorescent proteins, previously described for the earlier versions [21] . 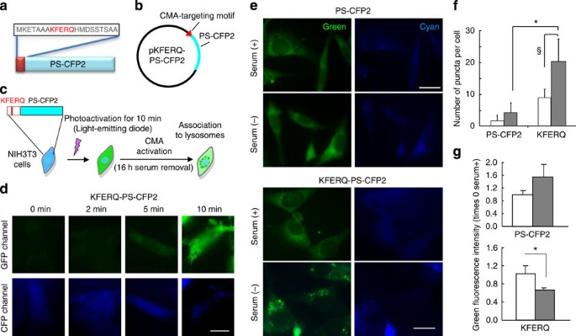Figure 1: The fluorescence pattern of the KFERQ–PS–CFP2 reporter changes during starvation. (a) Scheme of the insertion of the CMA-targeting motif in PS–CFP2. (b) Map of pKFERQ–PS–CFP2. (c) Scheme of the experimental design to monitor CMA activity in cultured cells using the KFERQ–PS–CFP2 reporter. (d) NIH3T3 cells stably expressing PS–CFP2 proteins were exposed to a 405 nm light for the indicated times and photoconverting was monitored by imaging cells in the green and blue channels. (e,f) Mouse fibroblasts (NIH3T3) stably expressing PS–CFP2 or KFERQ–PS–CFP2 were photoconverted and maintained in media supplemented (+) or not (−) with serum for 16 h. (e) Representative images in both channels. (f) Quantification of the number of green fluorescent puncta per cell in cells maintained in the presence (white bars) or absence (gray bars) of serum. Values are mean+s.e. of four different experiments with >50 cells counted per experiment. (*) Differences with PS–CFP2 in the green channel (P=0.005, ANOVA-Bonferroni). (§) Differences with samples in the presence of serum (P=0.03, ANOVA-Bonferroni). (g) Green fluorescence intensity at excitation 450 nm and emission 510–550 nm. Fluorescence intensity in each sample was normalized by the number of cells present in the sample and the percentage of intensity at time 0 still remaining after 16 h of incubation in the presence (white bars) or absence (gray bars) of serum was calculated for each condition. Values are expressed relative to the decay observed in cells maintained in the presence of serum and are means+s.e. of 3 independent experiments. Differences with serum (*) were significant forP=0.04 (t-test). Scale bars, 5 μm. Figure 1: The fluorescence pattern of the KFERQ–PS–CFP2 reporter changes during starvation. ( a ) Scheme of the insertion of the CMA-targeting motif in PS–CFP2. ( b ) Map of pKFERQ–PS–CFP2. ( c ) Scheme of the experimental design to monitor CMA activity in cultured cells using the KFERQ–PS–CFP2 reporter. ( d ) NIH3T3 cells stably expressing PS–CFP2 proteins were exposed to a 405 nm light for the indicated times and photoconverting was monitored by imaging cells in the green and blue channels. ( e , f ) Mouse fibroblasts (NIH3T3) stably expressing PS–CFP2 or KFERQ–PS–CFP2 were photoconverted and maintained in media supplemented (+) or not (−) with serum for 16 h. ( e ) Representative images in both channels. ( f ) Quantification of the number of green fluorescent puncta per cell in cells maintained in the presence (white bars) or absence (gray bars) of serum. Values are mean+s.e. of four different experiments with >50 cells counted per experiment. (*) Differences with PS–CFP2 in the green channel ( P =0.005, ANOVA-Bonferroni). (§) Differences with samples in the presence of serum ( P =0.03, ANOVA-Bonferroni). ( g ) Green fluorescence intensity at excitation 450 nm and emission 510–550 nm. Fluorescence intensity in each sample was normalized by the number of cells present in the sample and the percentage of intensity at time 0 still remaining after 16 h of incubation in the presence (white bars) or absence (gray bars) of serum was calculated for each condition. Values are expressed relative to the decay observed in cells maintained in the presence of serum and are means+s.e. of 3 independent experiments. Differences with serum (*) were significant for P =0.04 ( t -test). Scale bars, 5 μm. Full size image Excitation of mouse fibroblasts stably expressing KFERQ–PS–CFP2 with 405 nm light irreversibly photoconverts this recombinant protein from a cyan (excitation peak (ex) at 400 nm and emission peak (em) at 468 nm) to a green (ex. 490 nm and em. 511 nm) fluorescent state that can be easily tracked over the cyan background of the newly synthesized KFERQ–PS–CFP2 ( Fig. 1c ). On comparison of different types of photoactivation, we determined that 10 min photoactivation was enough to produce levels of conversion to green fluorescence, easily detected by fluorescence microscopy ( Fig. 1d ). Although some green fluorescent puncta could be identified in cells maintained in the presence of serum ( Fig. 1e ), removal of serum from the media for more than 10 h, a condition previously shown to result in activation of CMA [22] , changed the mostly diffuse green fluorescent pattern of KFERQ–PS–CFP2 to a punctate pattern, compatible with its association to lysosomes ( Fig. 1e ). In contrast, PS–CFP2 lacking the CMA-targeting motif maintained, for the most part, a diffuse cytosolic pattern. Quantification revealed a significant increase in the number of fluorescent KFERQ–PS–CFP2 puncta per cell in the serum-deprived cells ( Fig. 1f ), which is also significantly higher than the one observed for PS–CFP2, probably resulting from its 'in bulk' delivery to lysosomes by other forms of autophagy. As an alternative approach to quantify the lysosomal internalization of PS–CFP2 and KFERQ–PS–CFP2, we monitored the changes in total cellular green fluorescence intensity, which will decrease as the protein is internalized and degraded in this compartment. The higher reduction in the green fluorescence intensity on removal of serum in cells transfected with KFERQ–PS–CFP2, compared with cells incubated in the presence of serum, supports its enhanced degradation under these conditions ( Fig. 1g ). In contrast, in cells expressing PS–CFP2, serum removal did not accelerate the decay of green fluorescence over that observed in the presence of serum ( Fig. 1g ). Analysis of the fluorescence changes during a 30 h time course revealed a gradual increase in the number of fluorescent puncta ( Fig. 2a,b ) and a concomitant faster decrease in the intensity of green fluorescence ( Fig. 2c ) when serum was removed. In contrast, although cyan fluorescence decreased right after photoconversion, levels of this fluorescence were recovered within one hour and remained relatively constant afterwards ( Fig. 2d ). The stable levels of cyan fluorescence indicated that the degraded cyan protein was replaced by de novo synthesized protein that will also be blue ( Fig. 2d ). Overall, these studies support that the kinetics of CMA activation are similar to those described for these cells in in vitro systems using isolated lysosomes [11] . 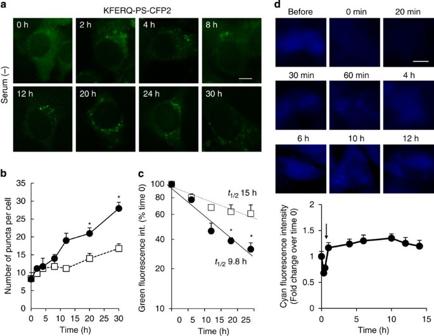Figure 2: Temporal course of the changes in KFERQ–PS–CFP2 fluorescence during starvation. (a–c) Temporal changes in the green fluorescence pattern of photoactivated NIH3T3 cells stably expressing KFERQ–PS–CFP2 maintained in the absence (black circles) or presence (white squares) of serum for the indicated times. (a) Representative images of cells maintained in serum-free media. Quantification of the number of puncta per cell (b) and green fluorescence intensity (c). Values are expressed as percentage of fluorescence at time 0 and half-lives (t1/2) are indicated. Differences in the number of puncta and fluorescence intensity between cells maintained in the presence and absence of serum (*) were significant forP=0.048 (16 h) andP=0.04 (24 h) (t-test). (d) The same cells imaged in the cyan channel, before and at the indicated times after photoconversion (arrow) by exposure to 405 nm light. Top: Representative images of the cyan fluorescence. Bottom: Quantification of the intensity of the cyan fluorescence. Values are expressed as times the intensity before photoconversion that was given an arbitrary value of 1. Values are mean+s.e. of 3 different experiments with >10 cells counted per experiment. Scale bars, 5 μm. Figure 2: Temporal course of the changes in KFERQ–PS–CFP2 fluorescence during starvation. ( a – c ) Temporal changes in the green fluorescence pattern of photoactivated NIH3T3 cells stably expressing KFERQ–PS–CFP2 maintained in the absence (black circles) or presence (white squares) of serum for the indicated times. ( a ) Representative images of cells maintained in serum-free media. Quantification of the number of puncta per cell ( b ) and green fluorescence intensity ( c ). Values are expressed as percentage of fluorescence at time 0 and half-lives ( t 1/2 ) are indicated. Differences in the number of puncta and fluorescence intensity between cells maintained in the presence and absence of serum (*) were significant for P =0.048 (16 h) and P =0.04 (24 h) ( t -test). ( d ) The same cells imaged in the cyan channel, before and at the indicated times after photoconversion (arrow) by exposure to 405 nm light. Top: Representative images of the cyan fluorescence. Bottom: Quantification of the intensity of the cyan fluorescence. Values are expressed as times the intensity before photoconversion that was given an arbitrary value of 1. Values are mean+s.e. of 3 different experiments with >10 cells counted per experiment. Scale bars, 5 μm. Full size image Association of the CMA reporter to lysosomes After activation of CMA by serum removal, most of the fluorescent puncta observed in cells expressing the KFERQ–PS–CFP2 was detected in acidic cellular compartments, highlighted with the pH-sensitive fluorophore LysoTracker ( Fig. 3a,b ). The high level of co-localization of KFERQ–PS–CFP2 with the lysosome-associated membrane proteins LAMP-1 and LAMP-2 supported the association of the CMA reporter with lysosomes ( Fig. 3b,c ). The fact that KFERQ–PS–CFP2 fluorescence was visible in the acid vesicles further supports that, as all other CMA substrates, the reporter protein was binding at the cytosolic side of the lysosomal membrane, because, once unfolded and translocated inside the lysosomal lumen, it will no longer be visible. The lower co-localization observed when, instead of the antibody against the luminal region of LAMP-2, we used an antibody against the cytosolic tail of the LAMP-2A variant—identified as the site of substrate binding in this CMA receptor [6] —likely reflects the inability of this antibody to recognize LAMP-2A proteins containing the KFERQ–PS–CFP2 bound to their cytosolic tail. 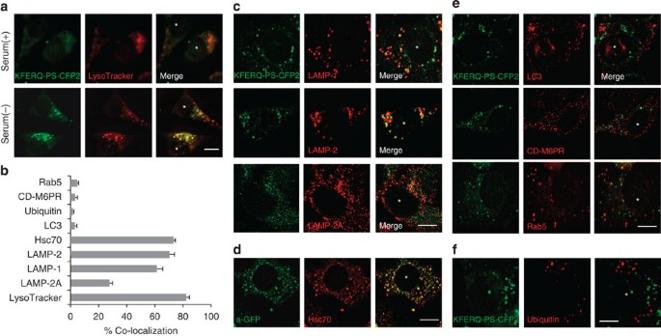Figure 3: KFERQ–PS–CFP2 co-localizes with lysosomes after induction of CMA. (a) Localization of photoconverted KFERQ–PS–CFP2 (green) in LysoTracker-stained compartments (red) in mouse fibroblasts maintained in the presence or absence of serum. (b) Percentage of co-localization of KFERQ–PS–CFP2 with the indicated proteins. Values are mean+s.e. of three different experiments with >50 cells counted per experiment. (c) Co-localization of photoconverted KFERQ–PS–CFP2 (green) with LAMP-1, LAMP-2 or LAMP-2A. (d) Immunofluorescence with antibodies that recognize PS–CFP2 (green) and hsc70 (red) in cells maintained in the absence of serum and fixed with methanol to eliminate the soluble cytosolic fraction. (e,f) Co-localization of photoconverted KFERQ-PS-CFP2 (green) with LC3, CD-M6PR, Rab5 (e) and ubiquitin (f) in mouse fibroblasts maintained in serum-free media. Scale bars, 5 μm. Figure 3: KFERQ–PS–CFP2 co-localizes with lysosomes after induction of CMA. ( a ) Localization of photoconverted KFERQ–PS–CFP2 (green) in LysoTracker-stained compartments (red) in mouse fibroblasts maintained in the presence or absence of serum. ( b ) Percentage of co-localization of KFERQ–PS–CFP2 with the indicated proteins. Values are mean+s.e. of three different experiments with >50 cells counted per experiment. ( c ) Co-localization of photoconverted KFERQ–PS–CFP2 (green) with LAMP-1, LAMP-2 or LAMP-2A. ( d ) Immunofluorescence with antibodies that recognize PS–CFP2 (green) and hsc70 (red) in cells maintained in the absence of serum and fixed with methanol to eliminate the soluble cytosolic fraction. ( e , f ) Co-localization of photoconverted KFERQ-PS-CFP2 (green) with LC3, CD-M6PR, Rab5 ( e ) and ubiquitin ( f ) in mouse fibroblasts maintained in serum-free media. Scale bars, 5 μm. Full size image Previous studies have revealed that CMA is carried out by a subset of lysosomes that contain in their lumen lys-hsc70, the chaperone required for substrate translocation [23] . To determine whether the CMA reporter associated to this subgroup of lysosomes, we fixed the KFERQ–PS–CFP2-expressing cells with methanol to eliminate most of the soluble cytosolic hsc70, preserving the one associated with organelles (CMA-active lysosomes, endosomes and endoplasmic reticulum). Using an antibody that recognizes PS–CFP2 (see Methods for details) to detect the reporter already translocated in the lysosomal lumen and no longer fluorescent, we found that ≥60% of vesicular structures positive for hsc70 also contained KFERQ–PS–CFP2 ( Fig. 3b,d ). These data, together with the co-localization with the other lysosomal constituent markers, supports that most of the KFERQ–PS–CFP2 visualized as fluorescent puncta were in CMA-active lysosomes. Although LAMPs can also be detected in autophagolysosomes and in late endosomes, in the conditions of our study, we did not observe co-localization of KFERQ–PS–CFP2 with LC3, a common marker for autophagic vacuoles, or with the mannose-6-phosphate receptor (CD-M6PR) or Rab5, markers of the late endocytic recycling compartment and early endosomes, respectively ( Fig. 3b,e ). The absence of co-localization with ubiquitin-positive puncta supported that the fluorescent puncta observed with KFERQ–PS–CFP2 did not result from mere aggregation of this protein ( Fig. 3b,f ). CMA delivers the photoswitchable reporter to lysosomes Although the fact that a high percentage of KFERQ–PS–CFP2 localized in the membrane of acidic vesicles positive for hsc70 supported its preferential association with CMA-active lysosomes, to conclusively determine whether most of the reporter reached lysosomes through CMA, we analysed changes in its distribution in cells incompetent for CMA. Interference against LAMP-2A (LAMP-2A (−)) has been shown to effectively prevent lysosomal delivery and degradation of proteins through CMA [11] . Fluorescence of KFERQ–PS–CFP2 expressed in LAMP-2A (−) cells remained, for the most part, as a diffuse cytosolic pattern, even after removal of serum ( Fig. 4a ). The failure to detect KFERQ–PS–CFP2 puncta in LAMP-2A (−) cells supports that this reporter requires functional CMA to reach lysosomes. In contrast, inhibition of macroautophagy, by treatment of cells with the PI3K inhibitor 3-methyladenine, did not have a significant effect in the number of KFERQ–PS–CFP2 positive vesicles detected in cells maintained in the presence or absence of serum ( Fig. 4b,c ). Consequently, the contribution of macroautophagy to the lysosomal delivery of KFERQ–PS–CFP2 is negligible. 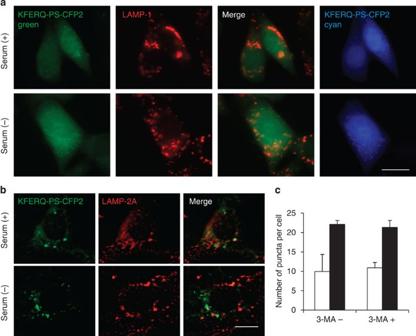Figure 4: Association of KFERQ–PS–CFP2 with lysosomes requires functional CMA. (a) Mouse fibroblasts knockeddown for LAMP-2A and transfected with KFERQ–PS–CFP2 were photoconverted and maintained in media supplemented (+) or not (−) with serum for 16 h. Representative images of cells also immunostained for LAMP-1 are shown. (b,c) Mouse fibroblasts stably expressing KFERQ–PS–CFP2 were photoconverted and maintained for 16 h in media supplemented (+) or not (−) with serum in the presence of 3-methyladenine (3-MA) to inhibit macroautophagy. (b) Representative images of the 3-MA-treated cells. (c) Quantification of the number of green fluorescence puncta per cell in 3-MA treated or not cells maintained in the presence (white bars) or absence (black bars) of serum. Values are mean+s.e. of 3 different experiments with >50 cells counted per experiment. No significant differences were detectable between samples supplemented or not with 3MA. Scale bars, 5 μm. Figure 4: Association of KFERQ–PS–CFP2 with lysosomes requires functional CMA. ( a ) Mouse fibroblasts knockeddown for LAMP-2A and transfected with KFERQ–PS–CFP2 were photoconverted and maintained in media supplemented (+) or not (−) with serum for 16 h. Representative images of cells also immunostained for LAMP-1 are shown. ( b , c ) Mouse fibroblasts stably expressing KFERQ–PS–CFP2 were photoconverted and maintained for 16 h in media supplemented (+) or not (−) with serum in the presence of 3-methyladenine (3-MA) to inhibit macroautophagy. ( b ) Representative images of the 3-MA-treated cells. ( c ) Quantification of the number of green fluorescence puncta per cell in 3-MA treated or not cells maintained in the presence (white bars) or absence (black bars) of serum. Values are mean+s.e. of 3 different experiments with >50 cells counted per experiment. No significant differences were detectable between samples supplemented or not with 3MA. Scale bars, 5 μm. Full size image To further confirm the association of the photoswitchable protein containing the CMA motif with lysosomes, we isolated lysosomes from mouse fibroblasts expressing PS–CFP2 and KFERQ–PS–CFP2 and subjected them to immunoblot ( Fig. 5 ). The fluorescent protein could not be detected in the membranes of lysosomes of cells expressing PS–CFP2 and only traces of the protein were observed in their matrix. In contrast, KFERQ–PS–CFP2 was detected both in membranes and in higher abundance in the lumens of isolated lysosomes ( Fig. 5a ). In agreement with the morphological data, the amount of KFERQ–PS–CFP2 was higher ( ∼ 3-fold increase) in lysosomes isolated from cells previously deprived of serum for >10 h ( Fig. 5b,c ), whereas the total cellular content of KFERQ–PS–CFP2 was about 30% less in cells maintained in the absence of serum ( Fig. 5b,d ; note that this decrease was lower than the 70% observed by direct fluorescence, because the signal in the immunoblot corresponds to both photoconverted and de novo synthesized KFERQ–PS–CFP2). Blockage of macroautophagy by treatment of cells with 3-methyladenine did not reduce the amount of KFERQ–PS–CFP2 detected in lysosomes ( Fig. 5e,f ), nor did it lead to an increase in total intracellular levels of KFERQ–PS–CFP2 ( Fig. 5g ). In fact, the slight increase in the content of KFERQ–PS–CFP2 in lysosomes isolated from 3-methyladenine-treated cells may reflect the compensatory upregulation of CMA in response to macroautophagy blockage described to occur in these cells [24] . 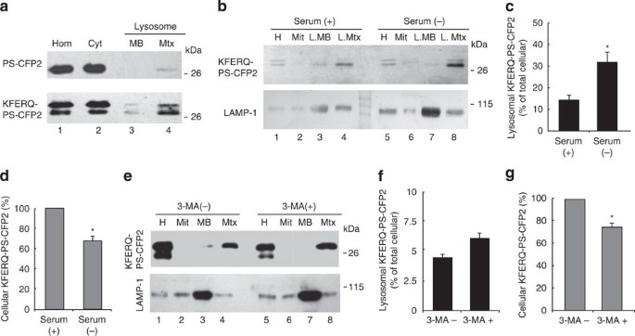Figure 5: KFERQ–PS–CFP2 proteins reach the lysosomal lumen. (a) Immunoblot with the antibody that recognizes PS–CFP2 of homogenates (Hom), cytosol (Cyt) and lysosomal membranes (MB) and matrices (Mtx) isolated from mouse fibroblasts stably expressing PS–CFP2 or KFERQ–PS–CFP2 proteins 16 h after serum removal. (b) Immunoblot for the indicated proteins of homogenates (Hom), mitochondria (Mit) and lysosomal membranes and matrices isolated from cells stably expressing KFERQ–PS–CFP2 maintained for 16 h in media supplemented (+) or not (−) with serum. (c) Quantification of the amount of KFERQ–PS–CFP2 associated to lysosomes (matrix and membrane) performed in blots as the one shown in (b). Values are expressed as percentage of the total KFERQ–PS–CFP2 in the cell and are mean+s.e. of three different experiments. Difference in the lysosomal associated KFERQ–PS–CFP2 between serum+ and serum− condition (*) were significant forP=0.033 (t-test). (d) Changes in the intracellular content of KFERQ–PS–CFP2 on serum removal. Values are expressed as percentage of KFERQ–PS–CFP2 present in serum-supplemented cells and area mean+s.e. of three different experiments. Values are mean+s.e. of three different experiments and differences are significant (*) forP=0.007 (t-test). (e–g) Effect of inhibition of macroautophagy by treatment with 3-methyladenine (3-MA) on the lysosomal content of KFERQ–PS–CFP2 in cells maintained in serum-free media for 16 h. (e) Immunoblot for the indicated proteins of the same fractions as described in (b). The amount of KFERQ–PS–CFP2 associated to lysosomes (f) and the changes in the intracellular content of KFERQ–PS–CFP2 were calculated as in (c,d). Values are mean+s.e. of three different experiments and differences are significant (*) forP=0.032 (t-test). Figure 5: KFERQ–PS–CFP2 proteins reach the lysosomal lumen. ( a ) Immunoblot with the antibody that recognizes PS–CFP2 of homogenates (Hom), cytosol (Cyt) and lysosomal membranes (MB) and matrices (Mtx) isolated from mouse fibroblasts stably expressing PS–CFP2 or KFERQ–PS–CFP2 proteins 16 h after serum removal. ( b ) Immunoblot for the indicated proteins of homogenates (Hom), mitochondria (Mit) and lysosomal membranes and matrices isolated from cells stably expressing KFERQ–PS–CFP2 maintained for 16 h in media supplemented (+) or not (−) with serum. ( c ) Quantification of the amount of KFERQ–PS–CFP2 associated to lysosomes (matrix and membrane) performed in blots as the one shown in ( b ). Values are expressed as percentage of the total KFERQ–PS–CFP2 in the cell and are mean+s.e. of three different experiments. Difference in the lysosomal associated KFERQ–PS–CFP2 between serum+ and serum− condition (*) were significant for P =0.033 ( t -test). ( d ) Changes in the intracellular content of KFERQ–PS–CFP2 on serum removal. Values are expressed as percentage of KFERQ–PS–CFP2 present in serum-supplemented cells and area mean+s.e. of three different experiments. Values are mean+s.e. of three different experiments and differences are significant (*) for P =0.007 ( t -test). ( e – g ) Effect of inhibition of macroautophagy by treatment with 3-methyladenine (3-MA) on the lysosomal content of KFERQ–PS–CFP2 in cells maintained in serum-free media for 16 h. ( e ) Immunoblot for the indicated proteins of the same fractions as described in ( b ). The amount of KFERQ–PS–CFP2 associated to lysosomes ( f ) and the changes in the intracellular content of KFERQ–PS–CFP2 were calculated as in ( c , d ). Values are mean+s.e. of three different experiments and differences are significant (*) for P =0.032 ( t -test). Full size image Both morphological and biochemical procedures confirm that KFERQ–PS–CFP2 is delivered to lysosomes through CMA, and that the abundance of this protein in the lysosomal compartment increases when this pathway is activated, such as during nutrient deprivation. Consequently, we propose that KFERQ–PS–CFP2 can be used to monitor CMA activity in these cells. Practical application of the KFERQ–PS–CFP2 reporter To determine whether the photoconvertible fluorescent reporter can be used to monitor CMA activity in different cell types, we transiently transfected cell lines of different origin with this reporter. 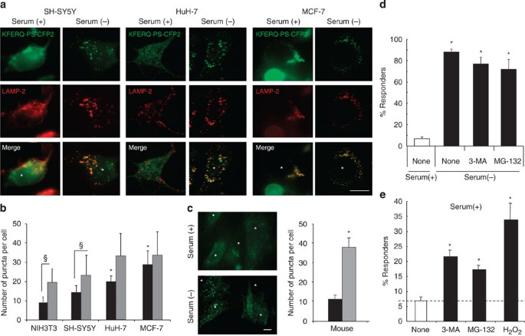Figure 6: Practical application of the KFERQ–PS–CFP2 reporter protein to monitor changes in CMA activity. (a,b) Human neuroblastoma (SH-SY5Y), hepatoma (HuH-7) and breast adenocarcinoma (MCF-7) cell lines were transiently transfected with KFERQ–PS–CFP2, photoconverted and maintained in media supplemented (+) or not (−) with serum for 16 h. Images show representative cells after immunostaining for LAMP-2 (red). (b) Quantification of the number of green fluorescent puncta per cell under basal conditions (black bars) and after serum removal (gray bars). Values of NIH3T3 are included as reference. Values are mean+s.e. of three-to-five different experiments with >50 cells counted per experiment. Differences with (*) NIH3T3 or (§) with cell supplemented with serum are significant forP<0.05 (range 0.002–0.03, ANOVA-Bonferroni). (c) Primary mouse skin fibroblasts were transduced with a lentiviral vector for expression of KFERQ–PS–CFP2, photoconverted and maintained in media supplemented (+) or not (−) with serum for 16 h. Left: representative image in the green channel. Right: Quantification of the number of green fluorescent puncta per cell in cells maintained in the presence (black bars) or absence (gray bars) of serum. Values are mean+s.e. of three different experiments with >50 cells counted per experiment. (P=0.002, ANOVA-Bonferroni). (d) Mouse fibroblasts stably expressing KFERQ–PS–CFP2 were plated in 384-well plates, maintained in the presence (white bar) or absence (black bars) of serum and subjected to treatment with 3-methyladenine (3-MA), the proteasome inhibitor MG-132 or H2O2. (e) Mouse fibroblasts stably expressing KFERQ–PS–CFP2 were plated in 384-well plates, maintained in the presence of serum supplemented media and leave untreated (white bar) or subjected to the indicated treatments (black bars). In both (d,e), after fixation, images were subjected to high content image analysis and the percent of responders was calculated in >200 cells per condition. Values are mean+s.e. of results in three different experiments. *P<0.001 (range 0.0002–0.0007,t-test). Scale bars, 5 μm. Figure 6a,b shows the presence of different number of KFERQ–PS–CFP2-positive puncta under basal conditions in human neuroblastoma, hepatoma and breast adenocarcinoma cell lines. This comparative analysis also revealed differences in the extent of the increase in number of fluorescent puncta in response to serum removal among cells. In fact, although both the hepatoma and breast adenocarcinoma cell lines display higher rates of basal CMA activity, they also have a proportionally reduced ability to further upregulate this pathway during nutritional compromise. Figure 6: Practical application of the KFERQ–PS–CFP2 reporter protein to monitor changes in CMA activity. ( a , b ) Human neuroblastoma (SH-SY5Y), hepatoma (HuH-7) and breast adenocarcinoma (MCF-7) cell lines were transiently transfected with KFERQ–PS–CFP2, photoconverted and maintained in media supplemented (+) or not (−) with serum for 16 h. Images show representative cells after immunostaining for LAMP-2 (red). ( b ) Quantification of the number of green fluorescent puncta per cell under basal conditions (black bars) and after serum removal (gray bars). Values of NIH3T3 are included as reference. Values are mean+s.e. of three-to-five different experiments with >50 cells counted per experiment. Differences with (*) NIH3T3 or (§) with cell supplemented with serum are significant for P <0.05 (range 0.002–0.03, ANOVA-Bonferroni). ( c ) Primary mouse skin fibroblasts were transduced with a lentiviral vector for expression of KFERQ–PS–CFP2, photoconverted and maintained in media supplemented (+) or not (−) with serum for 16 h. Left: representative image in the green channel. Right: Quantification of the number of green fluorescent puncta per cell in cells maintained in the presence (black bars) or absence (gray bars) of serum. Values are mean+s.e. of three different experiments with >50 cells counted per experiment. ( P =0.002, ANOVA-Bonferroni). ( d ) Mouse fibroblasts stably expressing KFERQ–PS–CFP2 were plated in 384-well plates, maintained in the presence (white bar) or absence (black bars) of serum and subjected to treatment with 3-methyladenine (3-MA), the proteasome inhibitor MG-132 or H 2 O 2 . ( e ) Mouse fibroblasts stably expressing KFERQ–PS–CFP2 were plated in 384-well plates, maintained in the presence of serum supplemented media and leave untreated (white bar) or subjected to the indicated treatments (black bars). In both ( d , e ), after fixation, images were subjected to high content image analysis and the percent of responders was calculated in >200 cells per condition. Values are mean+s.e. of results in three different experiments. * P <0.001 (range 0.0002–0.0007, t -test). Scale bars, 5 μm. Full size image In addition, insertion of the original CMA photoconvertible fluorescent reporter in the backbone of a lentiviral transfer vector allowed us to monitor the activity of this pathway in primary cell lines that are particularly difficult to transfect ( Fig. 6c shows primary skin fibroblasts). These studies confirm the universal applicability of this reporter across species and also reveal that basal levels of CMA and the intensity of the upregulation of this pathway in response to nutrient deprivation is cell-type-dependent. Lastly, we also analysed whether this novel CMA reporter could be adapted for use in high-content microscopy, a common readout method in high throughput screening nowadays. Removal of serum in mouse fibroblasts stably expressing KFERQ–PS–CFP2 and plated in a 384-well format significantly increased the percentage of responders (as defined under material and methods) ( Fig. 6d ). The increase in responders after serum removal was insensitive to blockage of macroautophagy or the proteasomal system. Using high-content microscopy analysis, we also validated that the KFERQ–PS–CFP2 reporter can be used to study upregulation of CMA in response to stimuli other than nutrient deprivation. Thus, we confirmed that blockage of macroautophagy under basal conditions results in increased CMA activity [24] and that this pathway is activated during oxidative stress [9] ( Fig. 6e ). In addition, we found that inhibition of proteasomal proteolysis, which did not have an effect on inducible CMA activity ( Fig. 6d ), increased basal CMA activity ( Fig. 6e ), unveiling that the cross-talk of CMA with other proteolytic pathways extends beyond the previously described interactions with macroautophagy. The molecular components behind this previously unknown compensatory activation of CMA during proteasome blockage are currently under investigation. We have validated the use of the CMA reporter to monitor the activity of this pathway in different types of cultured cells. In addition to the cell types shown here, this reporter has also been successfully used to monitor CMA in primary neuronal cultures, T cells, kidney tubular cells and adipocytes, supporting the universality of its application. However, we can foresee particular conditions in which the use of this reporter will need additional controls. For example, when used in cellular contexts favouring protein aggregation, some of the fluorescent puncta could result from aggregation of the KFERQ–PS–CFP2 reporter in cytosol. Positive co-localization with lysosomal markers should be used in this case to identify CMA-related puncta. Likewise, detection of the KFERQ–PS–CFP2-positive puncta and measurement of the decay of the green photoconverted reporter could be difficult in cells with high autofluorescent background or which accumulate autofluorescent pigment deposits, such as lipofuscin in ageing cells. To overcome this problem, we have developed a variation of the CMA reporter that consists of a KFERQ-bearing photoactivable mCherry protein, PA–mCherry1 [25] ( Fig. 7 ). KFERQ–PA–mCherry1 is initially non-fluorescent but fluoresces in red (ex. 564 nm and em. 595 nm) on irradiation using 405 nm light, allowing visualization of lysosomes as red fluorescent puncta, when CMA is activated ( Fig. 7a,b ). The fluorescent properties of the KFERQ–PA–mCherry1 reporter make it also suitable for analysis through fluorescence-activated cell sorting (FACS). 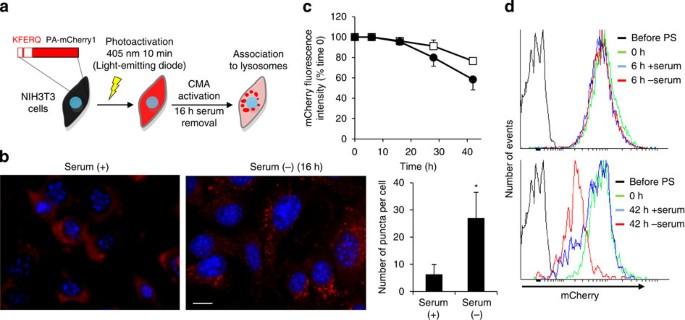Figure 7: A photoactivable fluorescent CMA reporter. (a) Scheme of the experimental design to monitor CMA activity in cultured cells using the KFERQ–PA–mCherry1 reporter. (b) Mouse fibroblasts (NIH3T3) stably expressing KFERQ–PA–mCherry1 were photoactivated and maintained in media supplemented (+) or not (−) with serum for 16 h. Left: Representative images. Nuclei are staining with DAPI. Right: Quantification of the number of red fluorescent puncta per cell. Values are mean+s.e. of three different experiments with >20 cells counted per experiment. *P=0.001, ANOVA-Bonferroni. (c) Temporal changes in the mCherry fluorescent intensity in cells stably expressing KFERQ–PA–mCherry1 at the indicated times after photoactivation using FACS analysis. Cells were maintained in media supplemented (white squares) or not (black circles) with serum, and fluorescence by the MFI was calculated on events gated on living cells. Values are expressed as percentage of the intensity at time 0 and are mean+s.e. of 3–4 individual experiments. (d) Representative FACS experiment showing the effect of serum removal at 6 h (top) and 42 h (bottom). PS, photoswitching. Scale bars, 5 μm. As shown in Figure 7c,d, measurement of the fluorescence intensity by FACS at different times after photoactivation in cells expressing the KFERQ–PA–mCherry1 reporter revealed a gradual decay in fluorescence that was accelerated in cells incubated in the absence of serum ( Fig. 7c,d ). FACS analysis may be a good alternative method for tracking CMA activity using the novel reporters in cells non-suitable for morphometric analysis by fluorescence microscopy (that is, cells undergoing changes in shape that prevent individual identification of fluorescent puncta). Figure 7: A photoactivable fluorescent CMA reporter. ( a ) Scheme of the experimental design to monitor CMA activity in cultured cells using the KFERQ–PA–mCherry1 reporter. ( b ) Mouse fibroblasts (NIH3T3) stably expressing KFERQ–PA–mCherry1 were photoactivated and maintained in media supplemented (+) or not (−) with serum for 16 h. Left: Representative images. Nuclei are staining with DAPI. Right: Quantification of the number of red fluorescent puncta per cell. Values are mean+s.e. of three different experiments with >20 cells counted per experiment. * P =0.001, ANOVA-Bonferroni. ( c ) Temporal changes in the mCherry fluorescent intensity in cells stably expressing KFERQ–PA–mCherry1 at the indicated times after photoactivation using FACS analysis. Cells were maintained in media supplemented (white squares) or not (black circles) with serum, and fluorescence by the MFI was calculated on events gated on living cells. Values are expressed as percentage of the intensity at time 0 and are mean+s.e. of 3–4 individual experiments. ( d ) Representative FACS experiment showing the effect of serum removal at 6 h (top) and 42 h (bottom). PS, photoswitching. Scale bars, 5 μm. Full size image Advances in the identification of the molecular mechanisms behind different autophagic pathways during recent years and the increasing number of connections between autophagic dysfunction and disease have generated growing interest in the study of autophagy. One of the major reasons why the study of CMA has been limited for years to only a handful of groups has been due to the fact that this autophagic pathway could only be monitored using specialized techniques that are not routine in most laboratories. Until now, the best method to determine changes in CMA activity has been by measuring the ability of isolated lysosomes to take up well-characterized CMA substrates [16] . CMA activity has only been indirectly inferred in cells through the combination of different approaches, which include, among others, metabolic radiolabelling and measurement of protein degradation in the presence of different protease inhibitors, and tracking of the number and intracellular localization of the subset of lysosomes active for CMA [16] . The genetically encoded photoconvertible PS–CFP2-based reporter described in this work should make monitoring of CMA in cells in culture broadly accessible and allow tracking the activity of this autophagic pathway in primary non-dividing cells, from which isolation of lysosomes is not feasible. Accumulation of tagged constitutive fluorescent proteins on blockage of proteolysis has been extensively used to investigate the activity of the ubiquitin/proteasome system and macroautophagy. Using photoconvertible proteins allows similar analysis without having to block protein synthesis and degradation [18] , [19] . An added advantage of photoconversion in the case of the CMA reporter is that it permits detection of the protein associated to the cytosolic side of the lysosomal membrane (green) against the cytosolic pool that, for the most part, is in a different fluorescence state (cyan). Furthermore, the use in our study of the new generation of fluorescent proteins (CFP, mCherry) that preserve their monomeric characteristics inside the cells [17] has helped in eliminating problems that could result from oligomerization of fluorescent proteins. This was particularly important, because it has been previously reported that protein oligomers formed by GFP-like proteins, such as DsRed and mRFP1, can be delivered to lysosomes, probably by macroautophagy- or microautophagy-related mechanisms [21] . We are confident that macroautophagy does not contribute significantly to the lysosomal association of our fluorescent reporter because, as shown in Figures 4c and 5f , blockage of macroautophagy did not have any significant effect on the amount of KFERQ–PS–CFP2 associated with lysosomes. Regarding microautophagy, we have recently reported that, in mammals, this process occurs preferentially in endosomes and it is independent of the presence of LAMP-2A [26] . However, the fact that we did not observe co-localization of KFERQ–PS–CFP2 with endosomes ( Fig. 3 ) and that knockdown of LAMP-2A effectively eliminated its association with lysosomes ( Fig. 4 ) makes contribution of microautophagy unlikely and supports that this novel reporter is delivered as monomers to lysosomes by CMA. KFERQ–PS–CFP2 does not co-localize completely with classic lysosomal markers such as LAMP-1 and LAMP-2; this is likely because these LAMPs are also present in endosomes (where CMA does not occur), and that not all cellular lysosomes are capable to perform CMA (although they all contain LAMPs), The unusually low level of co-localization of KFERQ–PS–CFP2 with LAMP-2A-positive structures could be explained by the same reasons as above, but in addition by the fact that the antibody used to differentiate the LAMP-2A variant from the other LAMP-2 proteins binds the same region as the CMA substrates (the 12 amino acids of the cytosolic tail). Therefore, staining for LAMP-2A will be lower when KFERQ–PS–CFP2 is bound to its cytosolic tail, as a result of activation of CMA. Previous analysis of KFERQ-containing proteins in different organs by immunoblot have revealed organ-specific differences in the abundance of these proteins during starvation, leading to proposed possible cell-type-dependent differences in CMA activity [27] . However, direct comparison of CMA activity across different cell types has not been possible until now. Our studies with the photoconvertible CMA reporters reveal that, indeed, the ability of cells to upregulate CMA in response to serum removal varies depending on the cell type. Furthermore, we have found that their basal CMA levels are also different. Future follow-up of these findings may help elucidate whether differences in the normal contribution of CMA to protein turnover among neuronal types is the reason behind their different susceptibility to blockage of this pathway by pathogenic proteins as is the case, for example, in Parkinson's disease. The coexistence of different proteolytic pathways inside cells and the fact that some proteins can undergo degradation by several of them support that, although not redundant, these pathways can compensate for each other. Indeed, previous studies have revealed the existence of a cross-talk between the two stress-induced forms of autophagy—macroautophagy and CMA—and between macroautophagy and the ubiquitin/proteasome system. Through the use of the photoconvertible reporters, we have now identified a new point of interaction between CMA and the proteasome. The ability to monitor CMA activity in intact cells makes it now possible to start addressing the issues whether this cross-talk is universal, the duration of the compensatory activations, and whether the ability to upregulate CMA or not, in pathological conditions with compromised proteasome activity, determines the rate of disease progression. Overall, as for any other image-based procedures, the use of the photoconvertible CMA reporters would be maximally strengthened by performing kinetic, rather than single-point analysis, and applying rigorous morphometric procedures. In addition, when used for the first time in a new cell type or under specific conditions, it is highly advisable to include the following controls in a pilot assay before the experimental analysis: checking for autofluoescence in untransfected cells; determining the kinetics of expression of the reporter (in the case of studies with transiently transfected cells); analysing the efficiency of photoconversion under the standard conditions described here and optimizing these parameters for the specific cell type, if needed; and analysing of cell viability after photoconversion (to determine possible toxic effect of the 405 nm light on specific cell types). We also recommend the following approach to validate that the formation of fluorescent puncta with the CMA reporter results indeed from the delivery of the fluorescent protein to lysosomes by this pathway: confirming that the puncta correspond to lysosomal location (by co-localizing with LysoTracker or lysosomal components such as LAMPs); discarding contribution of macroautophagy to the lysosomal delivery (by demonstrating absence of co-localization with LC3 or lack of effect of treatment with 3-methyl adenine in the final number of puncta); and confirming the dependence of the punctate pattern on CMA (by demonstrating absence of fluorescent puncta in LAMP-2A-deficient cells). In summary, we have developed a photoconvertible fluorescent reporter that allows monitoring and quantifying CMA activity in both transformed and primary cells in culture and have validated its applicability for high-content microscopy. Antibodies and reagents The antibody against LAMP-1 (clone 1D4B) (1 μg ml −1 ), the luminal region of LAMP-2 (1.4 μg ml −1 ) and against CD-M6PR (2 μg ml −1 ) were from the Developmental Hybridoma Bank (University of Iowa), against hsc70 (clone 13D3) (10 μg ml −1 ) and light chain 3 protein (LC3) (2.4 μg ml −1 ) from Novus Biotechnology, against Rab5 (clone D-11) (2 μg ml −1 ) from Santa Cruz Biotechnology and against ubiquitin from Zymed (clone Ubi-1) (2.5 μg ml −1 ). The polyclonal antibody raised against the enhanced green fluorescent protein (Sigma) was used at 0.4 μg ml −1 to recognize PS-CFP2 (both proteins have 88% sequence identity). The antibody against the cytosolic tail of LAMP-2A was developed in our laboratory [6] . LysoTracker Red DND 99 (100 nM) was from Invitrogen (Molecular Probes). Cell lines Mouse fibroblasts (NIH3T3), human neuroblastoma (SH-SY5Y), human hepatocarcinoma cells (HuH-7) and human breast adenocarcinoma (MCF-7) cell lines were from the American Type Culture Collection. Primary mouse fibroblasts were prepared in our laboratory following standard procedures. All animal work was approved and performed according to the guidelines set by the Albert Einstein College of Medicine Institutional Animal Care and Use Committee. LAMP-2A-knockdown cells were established by using vector-mediated stable RNA interference (RNAi) directed specifically against the LAMP-2A exon as described previously [11] . All cells were cultured in Dulbecco's Modified Eagle's Medium (DMEM) (Sigma) in the presence of 10% newborn calf serum or fetal bovine serum (FBS). Serum removal was performed by thoroughly washing the cells with Hanks' Balanced Salt Solution (Invitrogen) and placing them in serum-free complete medium. Where indicated, cells were treated with the macroautophagy inhibitor 3-methyladenine (Sigma) at a final concentration of 10 mM or with 100 μM leupeptin (Fisher BioReagents) to inhibit lysosomal proteolysis. Acid compartments were labelled in cultured cells by adding 100 nM LysoTracker in serum-free DMEM for 20 min. Construction of the reporter plasmids The pKFERQ–PS–CFP2 expression plasmid was constructed by inserting oligonucleotides coding for the sequence of 21 amino acids of ribonuclease A (MKETAAAKFERQHMDSSTSAA) (Accession number AAB35594) into the NheI and BamHI sites of a pPS–CFP2–N1 vector (Evrogen) ( Fig. 1a,b ). The oligonucleotides encoding for this 21 amino acids were as follows: 5′ ctagcgccaccatgaaggaaactgcagcagccaagtttgagcggcagcacatggactccagcacttccgctgcg 3′ and 5′ gatccgcagcggaagtgctggagtccatgtgctgccgctcaaacttggctgctgcagtttccttcatggtggcg 3′. The pKFEFQ–PA–mCherry1 plasmid was constructed by inserting the same fragment into the NheI and BamHI sites of the pPA–mCherry1-N1 vector [25] . To establish stable cell lines expressing the CMA reporter, pKFERQ–PS–CFP2-N1 or pPS-CFP2-N1 plasmids were transfected into NIH3T3 cells using lipofectamine2000 and selected with neomycin. Where indicated, the KFERQ–PS–CFP2 region was inserted between the blunt-ended BamHI and SalI sites of the pCCL.PPT.hPGK.GFP.Wpre lentiviral transfer vector [28] and lentiviral particles were generated by co-transfection with the third-generation packaging constructs pMDLg/pRRE and pRSV–REV, and as envelope the G glycoprotein of the VSV (pMD2.G) into HEK293T cells as described before. Photoconversion and imaging procedures Photoconversion of cells grown on coverslips was carried out with a 405/20 nm LED array (Norlux) for 10 min using 50 mW cm −2 light intensity. More than 90% of the cells were viable after the photoconversion. In the case of primary cultures, photoconversion time was reduced to 8 min to preserve >90% cell viability. For immunofluorescence, cells grown on coverslips were fixed in 3% formaldehyde in phosphate buffer saline (PBS), blocked with 10% FBS, permeabilized with 0.01% of TritonX-100 for 30 min, and then incubated with the primary and corresponding secondary antibodies diluted in 5% FBS in PBS. All images were acquired with an Axiovert 200 inverted fluorescence microscope (Zeiss) equipped with a ×63 1.4 NA oil objective lens and red (ex. 570/30 nm, em. 615/30 nm), cyan (ex. 365/50 nm and em. 530/45 nm) and green (ex. 475/40 nm and em. 535/45 nm) filter sets (Chroma). Acquired z-stack images were subjected to deconvolution using an Axio-Vision program (Zeiss) and then prepared using Adobe Photoshop 6.0 software (Adobe Systems). Quantification of co-localization was performed using Image J software (NIH) in individual frames after thresholding, and co-localization was calculated with the JACoP plugin of the same program in merged images. High-content microscopy analysis was performed in cells seeded in 384-well plates with transparent bottom and fixed as above but in the presence of Hoechst to stain nuclei. Fluorescence images were acquired and analysed using the ArrayScan HCS Reader (Thermo Scientific Cellomics). Fluorescence images in the green channel were produced using an ex. 475/40 nm, em. 535/45 nm filter set. Cell bodies were identified after Hoechst staining using an ex. 365/50 nm, em. 535/45 nm filter set. All images were acquired with a high-resolution CCD camera, using a ×20 dry objective lens. A sufficient number of fields were acquired to analyse at least 200 cells per well. Images were analysed with the Cellomics software according to the manufacturer's protocols using the spot detector bioapplication. Briefly, objects were identified as cells, if they had valid nuclei and cell-body measurements based on size and fluorescence intensity. Acceptable ranges for these parameters were determined in preliminary studies using untreated cells from multiple cultures. To classify cells as responders, each valid object was sequentially tested against a set of thresholds, and the total fluorescent spot area per cell had to exceed the minimum value (as defined in control cells). The percentage of responders was calculated as the total number of responder cells in a well relative to the selected object count. Fluorescence decay analysis To quantify the decay of green fluorescence intensity in different experimental conditions, cells were plated to confluence in 24-well plate, subjected to photoconversion and then trypsinized and fixed with 3% formaldehyde at the desired times. Fluorescence was measured in a 150 μl cuvette using a FluoroMax-3 spectrofluorometer (Jobin Yvon). Decay of the photoconverted proteins was calculated as a decrease in the green fluorescence intensity normalized to the number of cells determined by counting in a hemocytometer. Fluorescent intensity at each time point was subtracted by autofluorescence in non-transfected cells. Biochemical procedures For the isolation of subcellular fractions from cells in culture, a crude fraction containing lysosomes and mitochondria was prepared after cell lysis by nitrogen cavitation and differential centrifugation (2,500 g for 15 min; 17,000 g for 10 min). This fraction was subjected to centrifugation in discontinuous density metrizamide/percoll gradients as previously described [29] . Lysosomal matrices and membranes were isolated after hypotonic shock and centrifugation at 150,000 g for 30 min. Protein concentration was determined by the Lowry method using bovine serum albumin as a standard [30] . After SDS–PAGE and immunoblotting, the proteins recognized by the specific antibodies were visualized by chemiluminescence methods (Renaissance, NEN-Life Science). Densitometric quantification of the immunoblotted membranes was performed using Image J software (NIH). FACS analysis Cells fixed with 3% formaldehyde at the indicated times after photoactivation were subjected to FACS. mCherry fluorescent intensity was normalized to the maximal intensity after photoactivation. Statistical analysis All numerical results are reported as mean+s.e., and represent data from a minimum of three independent experiments unless otherwise stated. We determined the statistical significance of the difference between experimental groups in instances of single comparisons by the two-tailed unpaired Student's t -test of the means with the Sigma Plot software (Jandel Scientific). In instances of multiple means comparisons, we used one-way analysis of variance (ANOVA) followed by the Bonferroni post-hoc test to determine statistical significance. How to cite this article: Koga, H. et al . A photoconvertible fluorescent reporter to track chaperone-mediated autophagy. Nat. Commun. 2:386 doi: 10.1038/ncomms1393 (2011).